The low-affinity complex of cytochromecand its peroxidase The complex of yeast cytochrome c peroxidase and cytochrome c is a paradigm of the biological electron transfer (ET). Building on seven decades of research, two different models have been proposed to explain its functional redox activity. One postulates that the intermolecular ET occurs only in the dominant, high-affinity protein–protein orientation, while the other posits formation of an additional, low-affinity complex, which is much more active than the dominant one. Unlike the high-affinity interaction—extensively studied by X-ray crystallography and NMR spectroscopy—until now the binding of cytochrome c to the low-affinity site has not been observed directly, but inferred mainly from kinetics experiments. Here we report the structure of this elusive, weak protein complex and show that it consists of a dominant, inactive bound species and an ensemble of minor, ET-competent protein–protein orientations, which summarily account for the experimentally determined value of the ET rate constant. Biological electron transfer (ET) reactions are essential for many vital cellular activities including oxidative phosphorylation and photosynthesis—two processes underlying the conversion of energy from food or sunlight into the chemical energy of adenosine triphosphate. The complex of yeast proteins cytochrome c (Cc) and cytochrome c peroxidase (CcP) is the paradigm for the study of biological ET. Located in yeast mitochondria, CcP is a haem enzyme, which reduces hydroperoxides using the electrons provided by its physiological partner Cc. The catalytic mechanism of H 2 O 2 reduction involves the formation of CcP compound I (CpdI), an intermediate oxidized two equivalents above the CcP(Fe 3+ ) resting state and containing the Fe(IV)=O haem oxyferryl and the W191 +· cation radical [1] , [2] . Subsequent CpdI reduction in two one-electron steps involves complex formation with ferrous Cc, intermolecular ET and the product dissociation. On the basis of a substantial body of experimental work (reviewed in refs 1 , 2 ), two contrasting models have been put forward to explain the ET activity. According to the first one [3] , [4] , [5] , [6] , the ET occurs only from the Cc bound at the high-affinity site of CcP as seen in the X-ray structure of the complex [7] . An alternative mechanism proposes the existence of multiple ET-active protein–protein orientations and postulates that the ET from the Cc bound to a low-affinity site is faster than that in the crystallographic orientation [8] , [9] , [10] , [11] . Since then, the structure and ET properties of the low-affinity Cc–CcP complex have been a matter of active interest and ongoing debate. The first conclusive evidence for the 2:1 Cc–CcP complex formation came from the studies of Hoffman and co-workers [8] , [9] , [10] , who followed triplet-state quenching of Zn-substituted CcP or Cc by varying concentrations of the respective redox partner. The observed, rather complex, kinetics were explained by a model postulating two non-interacting Cc-binding sites of markedly different affinities and ET properties. Because of the big ( ∼ 10,000-fold) difference in the Cc affinities for the two binding sites, biophysical characterization of the ternary complex turned out to be an exceedingly difficult task, requiring a highly sensitive technique with a large dynamic range to detect small binding effects at the low-affinity site in the presence of a much stronger, dominant signal from the high-affinity site. To the best of our knowledge, only two non-kinetic, equilibrium studies have presented strong evidence for formation of the 2:1 Cc–CcP complex. In their early potentiometric work, Mauk et al. [12] observed Cc binding to two CcP sites with different protonation properties and established that the ternary complex is salt sensitive, with the second binding event abolished at high ionic strength ( I ≥100 mM). Then, in a more recent calorimetry study, Morar and Pielak [13] reported the 2:1 binding in the Cc–CcP system stabilized by trisaccharide melezitose and showed that the CcP mutation D148A disrupts the ternary complex formation, suggesting that this residue might be part of the low-affinity site. Despite these efforts, the exact location of the low-affinity site remains unclear, its binding properties in the absence of the sugar uncertain and the structure of the low-affinity complex unknown. To resolve these unknowns, here we present a structural characterization of the elusive low-affinity complex in solution. Two crucial elements were integral to the success of this study—decoupling of the binding events at the two sites and the use of solution NMR spectroscopy, in particular paramagnetic NMR, to obtain the relevant structural information. To achieve the first goal, we blocked the high-affinity CcP site by crosslinking (CL) the partner proteins via an intermolecular disulfide bond. With an overall positional root mean squared deviation of 2.5 Å between C α atoms of the CcP(V197C)-Cc(A81C) product and the native Cc–CcP complex [14] , this site-specific, covalent CL is an excellent structural mimic of the high-affinity binding geometry. Thus, with the proteins locked in the nearly-native crystallographic orientation, this CL enables the study of the low-affinity Cc–CcP interaction in the absence of strong binding effects from the high-affinity site. To solve the structure of the CL–Cc complex, we used paramagnetic relaxation enhancement (PRE) NMR spectroscopy, a powerful technique for studying weak complexes of soluble proteins [15] , [16] , [17] , [18] and characterizing minor states in the interactions of membrane-associated and integral membrane proteins [19] , [20] . The PRE is caused by a dipolar interaction between a nucleus and the unpaired electron(s) of the paramagnetic center, either present in the native protein or introduced by bioconjugation techniques. Because of the large magnetic moment of an unpaired electron and the r −6 distance dependence, the PRE effect is long-range (extending up to 35 Å) and exquisitely sensitive to lowly populated species [21] , [22] . Manifested by the decrease in NMR signal intensities, and generally measured as differences in the transverse relaxation rates of protons in the paramagnetic sample and a diamagnetic reference, 1 H Γ 2 PREs can be used as restraints in subsequent structure calculations [21] , [22] . Here we present a structural analysis of the low-affinity Cc–CcP complex in solution and show that it consists of a dominant protein–protein orientation and an ensemble of minor binding geometries, populating electrostatically favourable regions of the interaction space. We obtain individual, microscopic binding constants for the two species and assess their ET properties. Judging from the large distances between the Cc and CcP redox centres, the dominant binding form is inactive in the intermolecular ET. At the same time, the conformational ensemble constituting the minor species contains multiple, ET-competent protein–protein orientations with short haem–haem separations. The calculated ET rate constant is in excellent agreement with the experimentally measured value, suggesting that the low-affinity complex accounts for the measured haem–haem ET activity. Our findings settle the long-standing debate on the nature of the low-affinity Cc–CcP interaction and provide mechanistic insights into the intermolecular ET process in this paradigmatic system. Synthesis and characterization of the disulfide CLs To prepare covalent, disulfide-linked Cc–CcP complexes, we adopted the experimental strategy of Otting and co-workers [23] , wherein one of the single-cysteine protein variants is activated by Ellman’s reagent and then reacted with the free thiol-bearing binding partner (see Methods). Purified from the reaction mixture by ion-exchange chromatography, the resulting covalent CL elutes in a single peak, well separated from those of other protein components ( Fig. 1a ). To ensure the highest purity of the final sample, only the central part of the CL elution peak was collected (highlighted in Fig. 1a ), leaving out protein fractions at the leading and trailing edges. Estimated by ultraviolet–visible spectrophotometry of the final [D, 15 N] V197C CcP–A81C Cc CL stock solution, the overall yield of CL was at least 85 %. (The actual value is expected to be higher as not all CL fractions were included in the analysis.) The CL yield achieved here is substantially higher than 25–40% reported for the original CL experiments of Pappa and Poulos [24] or >60 % estimated in their follow-up work [14] , both of which employed Cu 2+ -catalysed oxidation of protein thiols to promote the intermolecular disulfide formation. 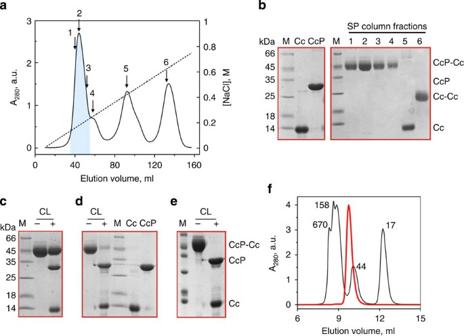Figure 1: Characterization of the [D,15N] V197C CcP–A81C Cc disulfide CL. (a) Purification of the CL by cation-exchange chromatography. The solid and dashed lines show the ultraviolet absorbance and the linear salt gradient (from 0 to 1 M NaCl in 20 mM NaPipH 6.0), respectively, for protein elution from a HiTrap SP FF column (GE Healthcare). Protein fractions analysed by SDS–PAGE are indicated by the arrows. The pooled fractions, containing the pure CL, are highlighted. (b) Non-reducing SDS–PAGE of reference samples (wt proteins) and the SP column fractions labelled ina. (c–e) SDS–PAGE with (+) and without (−) the disulfide reducing agent DTT of (c,d) the freshly purified CL and (e) the CL stock used for NMR experiments and stored for 1 month at 4 °C. Incubated for 15 min at room temperature, the ‘+’ sample in (c) contained 10 mM DTT, while those in (d,e) contained 125 mM DTT and were incubated for 15 min at 99 °C before analysis. For reference, the wt protein samples are included ind. Inb–e, ‘M’ denotes the molecular weight marker, with the values indicated on the left. (f) Analysis of the purified CL by analytical size-exclusion chromatography (SEC). Black and red lines show elution of the SEC protein standard (Bio-Rad) and the CL sample, respectively, from ENrich SEC 70 column (Bio-Rad) equilibrated in 20 mM NaPi0.1 M NaCl pH 6.0. The molecular weights (in kDa) of the reference proteins are indicated in the chromatogram. The expected molecular weight of the CL is 46 kDa. Figure 1: Characterization of the [D, 15 N] V197C CcP–A81C Cc disulfide CL. ( a ) Purification of the CL by cation-exchange chromatography. The solid and dashed lines show the ultraviolet absorbance and the linear salt gradient (from 0 to 1 M NaCl in 20 mM NaP i pH 6.0), respectively, for protein elution from a HiTrap SP FF column (GE Healthcare). Protein fractions analysed by SDS–PAGE are indicated by the arrows. The pooled fractions, containing the pure CL, are highlighted. ( b ) Non-reducing SDS–PAGE of reference samples (wt proteins) and the SP column fractions labelled in a . ( c – e ) SDS–PAGE with (+) and without (−) the disulfide reducing agent DTT of ( c , d ) the freshly purified CL and ( e ) the CL stock used for NMR experiments and stored for 1 month at 4 °C. Incubated for 15 min at room temperature, the ‘+’ sample in ( c ) contained 10 mM DTT, while those in ( d , e ) contained 125 mM DTT and were incubated for 15 min at 99 °C before analysis. For reference, the wt protein samples are included in d . In b – e , ‘M’ denotes the molecular weight marker, with the values indicated on the left. ( f ) Analysis of the purified CL by analytical size-exclusion chromatography (SEC). Black and red lines show elution of the SEC protein standard (Bio-Rad) and the CL sample, respectively, from ENrich SEC 70 column (Bio-Rad) equilibrated in 20 mM NaP i 0.1 M NaCl pH 6.0. The molecular weights (in kDa) of the reference proteins are indicated in the chromatogram. The expected molecular weight of the CL is 46 kDa. Full size image As shown in Fig. 1b–e , the [D, 15 N] V197C CcP–A81C Cc CL is highly pure and appears to be remarkably stable. In agreement with an earlier report [14] , treatment of this CL with 10 mM dithiothreitol (DTT) fails to reduce the intermolecular disulfide ( Fig. 1c ), which can be achieved only under strongly denaturing conditions with large amounts of the reducing agent ( Fig. 1d ). Stored at 4 °C, the CL stock solution remains stable for more than a month ( Fig. 1e ), a period of time largely sufficient for the NMR experiments conducted in this work. The two-dimensional (2D) [ 1 H, 15 N] transverse relaxation-optimized spectroscopy (TROSY) spectrum of [D, 15 N] V197C CcP(CN)–A81C Cc CL is highly similar to that of the free [D, 15 N] wild-type (wt) CcP(CN) [25] , enabling a facile transfer of backbone amide resonance assignments. The NMR signals of CcP residues 22–30 and 99–119, which are already weak in the free protein [25] , disappear in the CL, most likely because of a faster transverse relaxation caused by an increased rotational correlation time of the heavier CcP–Cc CL. In addition, the resonances of the CcP CL residues 193–199, located at the intermolecular interface, either disappear or shift to new spectral positions, which cannot be unambiguously assigned from an overlay of the two [ 1 H, 15 N] TROSY spectra. Overall, the high similarity of the NMR spectra of the free and Cc-linked CcP confirms that CL does not perturb the CcP molecule [14] and suggests that the individual proteins maintain their original structures, which justifies the rigid-body refinement of Cc–CcP complexes used in this and earlier works [26] , [27] , [28] . Similarly to the V197C CcP–A81C Cc CL discussed above, the other CLs used in this work can be obtained in high yield and purified to homogeneity ( Supplementary Figs 1 and 2 ). As established by SDS–PAGE (polyacrylamide gel electrophoresis) analysis, the final products correspond to the desired CLs. Represented by the sum of absorptions of individual proteins [29] , the ultraviolet–visible spectrum of a covalent complex ( Supplementary Fig. 1b ) confirms its purity and indicates that 3-thio-6-nitorbenzoate (TNB), used to activate cysteine residues during the CL reaction and featuring strong absorbance at 412 nm (ref. 30 ) does not co-purify with the protein samples. Chemical shift perturbation analysis Having prepared the protein CLs, we performed NMR chemical shift perturbation (Δ δ ) analysis of the CL–Cc interaction ( Fig. 2 ). To observe binding effects on both proteins, we monitored (1) the Cc complex formation with [D, 15 N] isotopically labelled, NMR-active CcP cross-linked to the natural-abundance, NMR-silent Cc and (2) binding of the NMR-active, 15 N-labelled Cc to the Cc–CcP CL in which both proteins are NMR-silent ( Fig. 2a,b , respectively). As seen in the [ 1 H, 15 N] correlation spectra of the 15 N-labelled proteins ( Fig. 2a,b ), stepwise addition of the binding partner leads to incremental shifts for several backbone amide resonances, indicating that the CL–Cc interaction is in fast exchange. Analysis of the CL- and Cc-observed NMR titration curves provided very similar values for the equilibrium dissociation constant ( K d ), suggesting that the effects observed from both protein sides report on the same binding event ( Fig. 2c,d ). The combined K d value of 2.0±0.4 mM obtained in this work is in good agreement with an earlier estimate, K d ≥1 mM, for the low-affinity binding under similar experimental conditions [12] . 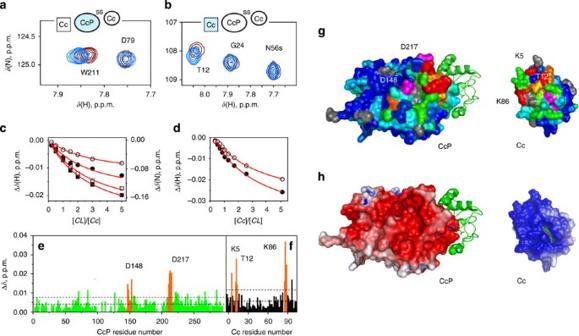Figure 2: Binding analysis of the low-affinity Cc–CcP complex. The CcP-observed Cc binding to the V197C CcP–A81C Cc CL and the Cc-observed binding of the CL in 20 mM NaPipH 6.0 at 25 °C. (a,b) Selected regions of the overlaid [1H,15N] heteronuclear single-quantum correlation spectra of the free proteins (blue) and in the presence of 5 equivalents of the corresponding binding partner (brown), showing typical chemical shift perturbations upon complex formation. The insets schematically depict the experimental set-up, with the NMR-active proteins coloured light blue. The symbol ‘s’ identifies a sidechain amide resonance. (c,d) NMR chemical shift titrations of (c) CL CcP nuclei A147 HN (open circles), D148 HN (filled circles), E214 HN (open squares) and L213 N (filled squares) and (d) Cc HN atoms of K86 (filled circles) and K5 (open circles). The curves in each plot were fitted simultaneously to a binding model with the sharedKd. The solid lines show the best fits with theKdvalues of 1.74±0.25 mM (CL-observed) and 2.30±0.66 mM (Cc-observed). (e,f) Binding-induced, combined chemical shift perturbations (Δδ) of the backbone amides of (e) CL CcP and (f) Cc. The horizontal lines indicate the average Δδand the average plus one standard deviation. Several clusters of residues most affected by the binding are indicated by the labels, with the Δδcoloured orange. (g) The Δδheat maps (coloured from 0.001 p.p.m. in blue to 0.02 p.p.m. in red; prolines and the residues with unassigned or unobserved backbone amide resonances are in grey) for the CL CcP and Cc. The labels indicate several residues affected by the binding. (h) Electrostatic properties of Cc and CcP, with molecular surfaces coloured by the electrostatic potential (from −5kBTin red to +5kBTin blue) calculated with APBS57. The molecular views ing,hshow X-ray structure of the Cc–CcP CL (PDB 1S6V)14with Cc as the green ribbon and CcP as the molecular surface and the Cc interface, with the haem group (g) coloured magenta or (h) shown in sticks. Figure 2: Binding analysis of the low-affinity Cc–CcP complex. The CcP-observed Cc binding to the V197C CcP–A81C Cc CL and the Cc-observed binding of the CL in 20 mM NaP i pH 6.0 at 25 °C. ( a , b ) Selected regions of the overlaid [ 1 H, 15 N] heteronuclear single-quantum correlation spectra of the free proteins (blue) and in the presence of 5 equivalents of the corresponding binding partner (brown), showing typical chemical shift perturbations upon complex formation. The insets schematically depict the experimental set-up, with the NMR-active proteins coloured light blue. The symbol ‘s’ identifies a sidechain amide resonance. ( c , d ) NMR chemical shift titrations of ( c ) CL CcP nuclei A147 HN (open circles), D148 HN (filled circles), E214 HN (open squares) and L213 N (filled squares) and ( d ) Cc HN atoms of K86 (filled circles) and K5 (open circles). The curves in each plot were fitted simultaneously to a binding model with the shared K d . The solid lines show the best fits with the K d values of 1.74±0.25 mM (CL-observed) and 2.30±0.66 mM (Cc-observed). ( e , f ) Binding-induced, combined chemical shift perturbations (Δ δ ) of the backbone amides of ( e ) CL CcP and ( f ) Cc. The horizontal lines indicate the average Δ δ and the average plus one standard deviation. Several clusters of residues most affected by the binding are indicated by the labels, with the Δ δ coloured orange. ( g ) The Δ δ heat maps (coloured from 0.001 p.p.m. in blue to 0.02 p.p.m. in red; prolines and the residues with unassigned or unobserved backbone amide resonances are in grey) for the CL CcP and Cc. The labels indicate several residues affected by the binding. ( h ) Electrostatic properties of Cc and CcP, with molecular surfaces coloured by the electrostatic potential (from −5 k B T in red to +5 k B T in blue) calculated with APBS [57] . The molecular views in g , h show X-ray structure of the Cc–CcP CL (PDB 1S6V) [14] with Cc as the green ribbon and CcP as the molecular surface and the Cc interface, with the haem group ( g ) coloured magenta or ( h ) shown in sticks. Full size image As seen in other NMR studies of such weak protein–protein interactions [17] , [18] , [31] , the chemical shift perturbations observed here are small ( Fig. 2a,b,e,f ), reflecting the modest equilibrium population of the Cc–CL complex in the NMR samples. The Δ δ analysis reveals that, for both proteins, the binding effects are confined to several clusters of residues constituting contiguous surface patches ( Fig. 2g ). Most of the affected CcP groups are found in the region bordering D148 and D217, identified in a classic Brownian dynamics study as the likely location of the low-affinity site [32] . On the Cc side, the binding interface is defined by K5, T12 and K86, encompassing an area adjacent to the exposed haem edge. Believed to be driven by complementary electrostatics, the low-affinity Cc–CcP interaction indeed appears to involve oppositely charged protein surfaces as demonstrated by the present NMR analysis and Poisson–Boltzmann calculations ( Fig. 2g,h ). Finally, our conclusions are reinforced by the control experiments showing that the Cc binding to CcP(E290C)-Cc(K73C) CL, an alternative mimic of the high-affinity complex, proceeds via essentially the same protein interface and with the same K d as those of the CL discussed above ( Supplementary Fig. 3 ). PRE NMR spectroscopy The Δ δ analysis provides good qualitative description of the Cc–CL binding interface, yet it is insufficient for establishing the mutual orientation of the binding partners, that is, the structure of the complex [33] . To obtain the quantitative structural information necessary to achieve this goal, we used PRE NMR spectroscopy. Here intermolecular PREs for the low-affinity Cc–CcP complex were obtained in essentially the same experimental set-up as that used in our recent study of the high-affinity Cc–CcP interaction [28] . In particular, three single-cysteine Cc variants D50C, E66C and E88C were labelled with an EDTA-based, chelating tag containing a paramagnetic metal ion (Mn 2+ , S =5/2), and their interactions with [D, 15 N] CcP cross-linked to the natural-abundance Cc were monitored in [ 1 H, 15 N] TROSY experiments. Following an established methodology [28] , a set of intermolecular PREs—detected on the CcP backbone amide protons—was obtained from a series of TROSY spectra, yielding distinct Γ 2 profiles for each Cc-EDTA(Mn 2+ ) variant ( Fig. 3a ). Driven by the combined set of Γ 2 restraints from all three EDTA(Mn 2+ ) positions, structure calculations of the Cc–CL complex produced a set of well-defined low-energy solutions ( Fig. 3b and Supplementary Fig. 4 ). Featuring Cc bound to the CcP face bordered by D148 and D217 residues, the low-affinity Cc–CcP-binding geometry is in excellent agreement with the chemical shift perturbation maps ( Fig. 3c , also compare Figs 3b and 2g ). This finding is even more striking as no Δ δ data were used in the molecular refinement. With the shortest distance of 19 Å between any two heavy atoms of the two cytochromes, there is no direct interaction between Cc molecules bound to the low- and high-affinity sites. 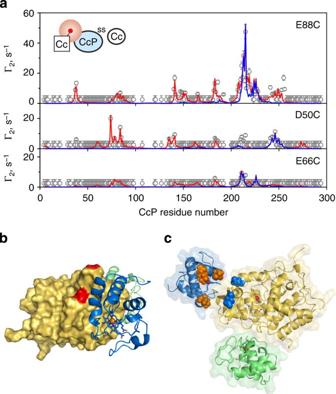Figure 3: Structure of the low-affinity Cc–CcP complex. (a) Intermolecular, CcP-observed PREs for the CL in the complex with Cc paramagnetically labelled at E88C, D50C, and E66C. The plots show measured PREs (open symbols), Γ2values back-calculated from the single, lowest-energy CL–Cc structure (blue line) and the PREs calculated for the combination of the dominant binding geometry and multiple protein–protein orientations obtained in a typical ensemble refinement run (red line). The errors are s.d. The inset schematically depicts the experimental set-up, with the NMR-active protein coloured light blue and the attached paramagnetic label indicated by the red sphere. (b) The structure of the dominant form of the CL–Cc complex. Cc bound to the low-affinity CcP site is shown as blue cartoon, while the CL CcP and Cc are represented as the yellow molecular surface and the green cartoon, respectively. The CL orientation is the same as inFig. 2g. CcP residues D148 and D217 are coloured red. Haem groups are shown as sticks, with iron atoms as spheres. (c) The intermolecular interface of the dominant low-affinity binding orientation. The proteins are coloured as inb. CcP residues D148 and D217 and Cc residues K5, T12 and K86 spacefilled and shown in blue and orange, respectively. Figure 3: Structure of the low-affinity Cc–CcP complex. ( a ) Intermolecular, CcP-observed PREs for the CL in the complex with Cc paramagnetically labelled at E88C, D50C, and E66C. The plots show measured PREs (open symbols), Γ 2 values back-calculated from the single, lowest-energy CL–Cc structure (blue line) and the PREs calculated for the combination of the dominant binding geometry and multiple protein–protein orientations obtained in a typical ensemble refinement run (red line). The errors are s.d. The inset schematically depicts the experimental set-up, with the NMR-active protein coloured light blue and the attached paramagnetic label indicated by the red sphere. ( b ) The structure of the dominant form of the CL–Cc complex. Cc bound to the low-affinity CcP site is shown as blue cartoon, while the CL CcP and Cc are represented as the yellow molecular surface and the green cartoon, respectively. The CL orientation is the same as in Fig. 2g . CcP residues D148 and D217 are coloured red. Haem groups are shown as sticks, with iron atoms as spheres. ( c ) The intermolecular interface of the dominant low-affinity binding orientation. The proteins are coloured as in b . CcP residues D148 and D217 and Cc residues K5, T12 and K86 spacefilled and shown in blue and orange, respectively. Full size image As can be seen in Fig. 3a , not all Γ 2 restraints are accounted for by the single Cc–CL structure. Observed before for the high-affinity Cc–CcP complex [26] , [28] —shown to comprise the dominant binding form and an ensemble of lowly populated protein–protein orientations sampled in the transient encounter state—such additional PREs are the footprint of minor species [21] , [22] . Unlike the chemical shift perturbation, which is a linear, population-weighted average of Δ δ s in different protein–protein orientations, PRE is an < r −6 >-dependent effect. Thus, if the electron–nucleus distance in the minor form is shorter than that in the dominant one, the former will give rise to a very large PRE, making a measurable contribution to the overall, population-weighted Γ 2 value [21] , [22] . This explains why additional effects, not present in the Δ δ plots, are observed in the Γ 2 profiles. As described in detail in our recent study of the high-affinity Cc–CcP complex, the EDTA(Mn 2+ ) conjugation to Cc yields a single, well-defined product and does not perturb the native Cc–CcP binding [28] . To ascertain that the PREs presented in Fig. 3a are not experimental artifacts, but indeed arise from the Cc–CL interaction, we performed a number of control experiments. First, we addressed a possible aspecific binding of the attached paramagnetic probe to the NMR-active protein, which is of particular concern under the low ionic strength conditions of the present study. As shown in Fig. 4a , the Cc interaction with paramagnetically labelled CcP gives rise to very strong PRE effects, affecting two protein regions (highlighted). Control experiments with the paramagnetically labelled ubiquitin (Ub)—an unrelated protein that binds neither Cc nor CcP—yield Γ 2 profiles with strong effects in the same two regions ( Fig. 4b ). Finally, Cc appears to bind the free EDTA(Mn 2+ ) probe as evidenced by large PREs affecting one of the aforementioned protein areas ( Fig. 4c ). Taken together, these findings reveal an undesired interaction between oppositely charged Cc and the CcP-tethered EDTA(Mn 2+ ) moiety, which precluded the Cc-observed NMR experiments with the paramagnetically labelled CcP, initially intended as part of this work. 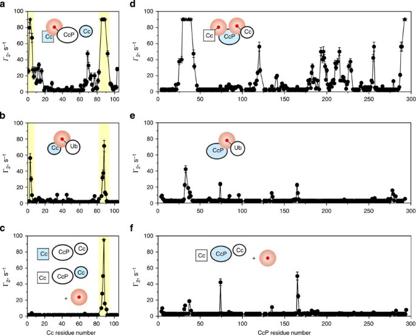Figure 4: PRE control experiments. Intermolecular PREs for the backbone amide resonances of (a–c)15N Cc caused by (a) CcP E221C-EDTA(Mn2+), (b) Ub D32C-EDTA(Mn2+) and (c) free paramagnetic label; and (d–f) [D,15N] wt CcP caused by (d) Cc E88C-EDTA(Mn2+), (e) Ub D32C-EDTA(Mn2+) and (f) free paramagnetic label. Stars indicate the residues whose resonances disappear in the paramagnetic spectrum. The errors are s.d. The insets schematically depict the experimental set-up, with the NMR-active protein coloured light blue and the paramagnetic label indicated by the red sphere. The Cc regions that experience strong PREs are highlighted. The NMR samples contained (a) 0.3 mM of CcP E221C-EDTA(Mn2+) and 3 equivalents of15N Cc; (b) 0.3 mM15N Cc and 3 equivalents of Ub D32C-EDTA(Mn2+); (c) 0.3 mM wt CcP, 0.45 mM each of15N-labelled and natural-abundance Cc, and 0.45 mM of the free paramagnetic label; (d) 0.4 mM [D,15N] wt CcP and 3 equivalents of Cc E88C-EDTA(Mn2+); (e) 0.4 mM [D,15N] wt CcP and 3 equivalents of Ub D32C-EDTA(Mn2+). The sample infwas generated from that indby addition of twofold molar excess (relative to Cc) of DTT, which breaks the disulfide bond between Cc and the EDTA(Mn2+) moiety, releasing the latter into the solution. All experiments were conducted in 20 mM NaPipH 6.0 at 25 °C. Figure 4: PRE control experiments. Intermolecular PREs for the backbone amide resonances of ( a – c ) 15 N Cc caused by ( a ) CcP E221C-EDTA(Mn 2+ ), ( b ) Ub D32C-EDTA(Mn 2+ ) and ( c ) free paramagnetic label; and ( d – f ) [D, 15 N] wt CcP caused by ( d ) Cc E88C-EDTA(Mn 2+ ), ( e ) Ub D32C-EDTA(Mn 2+ ) and ( f ) free paramagnetic label. Stars indicate the residues whose resonances disappear in the paramagnetic spectrum. The errors are s.d. The insets schematically depict the experimental set-up, with the NMR-active protein coloured light blue and the paramagnetic label indicated by the red sphere. The Cc regions that experience strong PREs are highlighted. The NMR samples contained ( a ) 0.3 mM of CcP E221C-EDTA(Mn 2+ ) and 3 equivalents of 15 N Cc; ( b ) 0.3 mM 15 N Cc and 3 equivalents of Ub D32C-EDTA(Mn 2+ ); ( c ) 0.3 mM wt CcP, 0.45 mM each of 15 N-labelled and natural-abundance Cc, and 0.45 mM of the free paramagnetic label; ( d ) 0.4 mM [D, 15 N] wt CcP and 3 equivalents of Cc E88C-EDTA(Mn 2+ ); ( e ) 0.4 mM [D, 15 N] wt CcP and 3 equivalents of Ub D32C-EDTA(Mn 2+ ). The sample in f was generated from that in d by addition of twofold molar excess (relative to Cc) of DTT, which breaks the disulfide bond between Cc and the EDTA(Mn 2+ ) moiety, releasing the latter into the solution. All experiments were conducted in 20 mM NaP i pH 6.0 at 25 °C. Full size image Unlike in the Cc case, the CcP-observed control experiments testify to the absence of significant aspecific interactions ( Fig. 4d–f ). The wt CcP binding to Cc-EDTA(Mn 2+ ) produces a Γ 2 profile featuring large PREs, most of which arise from the high-affinity Cc–CcP binding form and the associated encounter complex ( Fig. 4d ) [28] . At the same time, experiments with paramagnetically labelled Ub and the free EDTA(Mn 2+ ) show only a few weak effects ( Fig. 4e, f ), which are not found in the PRE profiles of either wt CcP or the CcP–Cc CL ( Figs 4d and 3a , respectively). Moreover, distinct CcP-detected PRE patterns are observed for CL complexes with different Cc-EDTA(Mn 2+ ) variants ( Fig. 3a ), which would be unlikely if the measured effects were dominated by the binding of the paramagnetic probe—expected to be largely insensitive to the attachment site. Finally, the intermolecular PREs observed in the CL–Cc system are reproducible ( Supplementary Fig. 5 ), and the CL–Cc Γ 2 effects are also detected in the native, non-covalent wt CcP–Cc complex (see below). These findings confirm that the measured PREs report on the Cc–CcP binding, and not a trivial protein-probe interaction. Structural and thermodynamic analysis of the minor species To estimate the population of the minor species and visualize the constituent protein–protein orientations, we performed conjoint refinement [34] of the dominant Cc–CL complex and an ensemble of additional binding forms against the observed PREs. In practice, the relative populations of the two bound species, p 1 and p 2 , were varied in multiple refinement runs. Each time, the agreement between the experimental data and the Γ 2 values back-predicted from the resulting solutions was evaluated by calculating the Q factor (equation 1)—a quantitative measure of the fit, with smaller Q values indicating a better match [34] . The plot in Fig. 5a shows Q as a function of p 1 and p 2 for two distinct binding scenarios. First, if the K d value of 2 mM obtained in this work is the total, macroscopic dissociation constant for the low-affinity complex ( K d,tot ), comprising both the dominant and minor species, then p 1 + p 2 =1. In this case, the overall amount of CL bound to Cc is independent of the relative populations of the two binding forms. In contrast, if the measured K d value is the microscopic dissociation constant for the dominant binding site only ( K d,1 ), then the fraction of bound CL rises with increasing p 2 (that is, p 1 + p 2 >1 at fixed p 1 =1). The results of molecular refinement corresponding to the two situations are presented in the left- and right-hand side plots of the Fig. 5a , respectively. The Q values in the right panel are consistently smaller than those on the left, with the minimal values located in the region of p 2 =0.6−0.9 at the constant p 1 =1.0 indicating the best agreement with the experimental data. Thus, comparative analysis of the Q factors allows to discriminate between the two binding scenarios. Moreover, the determined populations can be converted into the microscopic dissociation constants for the two binding forms, K d,1 =2.0±0.4 mM and K d,2 =2.7±0.5 mM, as well as the overall, macroscopic K d,tot =1.2±0.2 mM for the low-affinity complex ( Supplementary Note 1 and Supplemetary Fig. 7 ). As demonstrated in earlier studies [35] , [36] and mentioned above, chemical shift perturbations are largely insensitive to the presence of minor species comprising multiple, transient protein–protein orientations and report mainly on the dominant form of the complex. This explains why the Δ δ titrations performed here provided the microscopic dissociation constant for the dominant CL–Cc form only, as confirmed by the PRE-based Q -factor analysis. 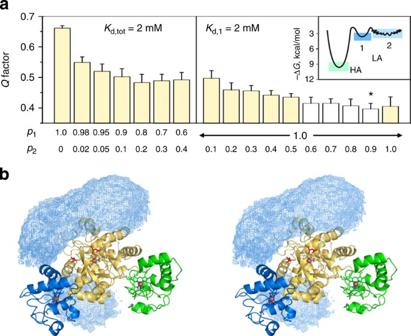Figure 5: Ensemble refinement of the lowly populated CL–Cc forms. (a)Qfactors for ensemble refinement of CL–Cc complexes at varying relative populations of the two bound species,p1andp2, and two binding scenarios (see text). White bars indicate the smallestQvalues. An asterisk identifies the data set presented inb. The inset shows a schematic energy diagram for the native, non-covalent Cc–CcP complex, where ‘HA’ and ‘LA’ refer to the high- and low-affinity domains, respectively, and ‘1’ and ‘2’ indicate the two binding sites of the latter (see text for details). (b) Stereo image showing Cc molecules in the dominant binding geometry (blue cartoon) and multiple minor forms of the low-affinity Cc–CcP complex, displayed as a reweighted atomic probability density map for the overall distribution of the Cc heavy atoms plotted at a threshold of 40% maximum58. The CL CcP and Cc are coloured yellow and green, respectively. Figure 5: Ensemble refinement of the lowly populated CL–Cc forms. ( a ) Q factors for ensemble refinement of CL–Cc complexes at varying relative populations of the two bound species, p 1 and p 2 , and two binding scenarios (see text). White bars indicate the smallest Q values. An asterisk identifies the data set presented in b . The inset shows a schematic energy diagram for the native, non-covalent Cc–CcP complex, where ‘HA’ and ‘LA’ refer to the high- and low-affinity domains, respectively, and ‘1’ and ‘2’ indicate the two binding sites of the latter (see text for details). ( b ) Stereo image showing Cc molecules in the dominant binding geometry (blue cartoon) and multiple minor forms of the low-affinity Cc–CcP complex, displayed as a reweighted atomic probability density map for the overall distribution of the Cc heavy atoms plotted at a threshold of 40% maximum [58] . The CL CcP and Cc are coloured yellow and green, respectively. Full size image The ensemble refinement of the minor Cc–CL form consistently produced solutions with bound Cc molecules populating two spatial regions: one bordering CcP residues D148 and D217 and extending to the surface patch containing D33 and E35, and the other defined by the CcP residues E167, D261 and E267 ( Fig. 5b ). Multiple Cc conformers of the minor species do not overlap with the Cc molecule in the dominant Cc–CL form, even though such overlap was allowed in the ensemble refinement protocol. This finding validates the present quantitative analysis of the low-affinity Cc–CL complex with the binding model for two individual, non-overlapping sites. Extending these conclusions to the native, non-covalent Cc–CcP complex, and borrowing the terminology of Hoffman and co-workers [11] , we can say that CcP harbours two domains—those binding Cc with high and low affinity and yielding, respectively, the crystallographic Cc–CcP form and the weak complex studied here. The low-affinity domain contains two binding sites comprising the dominant protein–protein orientation and an ensemble of lowly populated binding geometries, which summarily account for the observed PRE effects. Such dynamic view of the ternary CcP–(Cc) 2 complex agrees with conclusions of earlier computational studies and very recent ET kinetics work [32] , [37] . The equilibrium populations of different bound species, determined from microscopic K d s for the two low-affinity sites obtained in this work and the reported K d values for the high-affinity domain [1] , can be converted into the corresponding binding energies, schematically depicted in the energy diagram (inset in Fig. 5a ). Previous experimental studies suggested that electrostatic repulsion between two Cc molecules in the ternary complex accounts for the drastic difference in the affinity constants for the first and second binding steps [37] , [38] , [39] . Difference in binding energies for the high- and low-affinity sites (ΔΔ G ) provides the upper limit for the electrostatic repulsion energy (Δ G Φ ), a presumed dominant term in the energy penalty for such ‘anticooperative’ binding. The value of ΔΔ G ≤5.5 kcal mol −1 calculated in this work can be compared with those of Δ G Φ =6 kcal mol −1 and Δ G Φ ≤3.3 kcal mol −1 obtained from steady-state kinetics and flash photolysis experiments conducted under similar experimental conditions [37] , [39] . Experimental validation of the observed binding effects Analysis of the intermolecular PREs at different ionic strengths confirms that the Cc binding to the low-affinity CcP domain is salt sensitive ( Fig. 6 ). For most of the CL CcP residues, the paramagnetic effect decreases exponentially with the increasing salt concentration, yielding essentially flat Γ 2 profiles at 100 mM NaCl ( Fig. 6a, b ). Thus, in agreement with earlier studies [1] , [2] , [12] , the low-affinity binding is abolished at 100 mM salt. Consistent with this finding, the effects originating from the low-affinity domain account for most of the differences between the PRE profiles of the native, non-covalent Cc–CcP complex at high and low ionic strengths ( Fig. 7 ). At 100 mM NaCl, the measured PREs are well represented by a combination of effects from the high-affinity binding geometry and its transient encounter state ( Fig. 7a ) [28] . Reflecting the higher fraction of CcP bound, the corresponding Γ 2 values at 0 mM NaCl are consistently larger, but for the most part follow the same pattern as those at high ionic strength, suggesting that the structure of the Cc–CcP complex and its encounter state remains the same ( Fig. 7b ). Manifested as additional contributions to the low-salt PRE data, the main differences between the two Γ 2 profiles are found for the CcP regions that sense Cc binding to the low-affinity domain (highlighted in Fig. 7 ). These results show that the observed effects are not specific to the Cc–CL system, but are also found in the native, non-covalent complex. 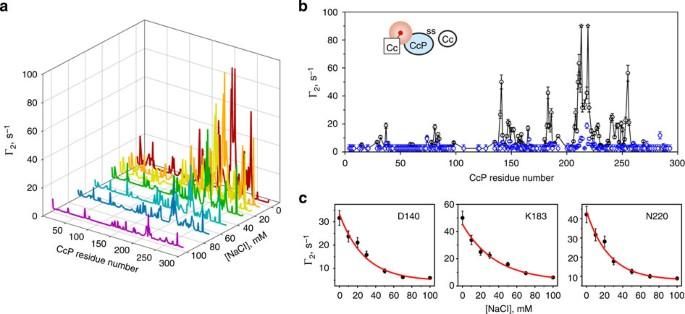Figure 6: Effect of the ionic strength on the intermolecular PREs in the CL–Cc system. (a) CcP-observed Γ2PREs for the CL in the presence of 3 equivalents of Cc E88C-EDTA(Mn2+) in 20 mM NaPipH 6.0 at varying concentrations of NaCl. (b) Comparison of the PRE profiles obtained at 0 mM (black) and 100 mM (blue) NaCl. Stars indicate the residues whose resonances disappear in the paramagnetic spectrum. The errors are s.d. The inset schematically depicts the experimental set-up, with the NMR-active protein coloured light blue, and the attached paramagnetic label indicated by the red sphere. (c) Ionic strength dependence of Γ2for several CL CcP residues. The errors are s.d. The red lines show the best fits to an exponential decay function with the decay rates of 28±4 (D140,r2=0.97), 36±6 (K183,r2=0.98) and 25±4 (N220,r2=0.98). Figure 6: Effect of the ionic strength on the intermolecular PREs in the CL–Cc system. ( a ) CcP-observed Γ 2 PREs for the CL in the presence of 3 equivalents of Cc E88C-EDTA(Mn 2+ ) in 20 mM NaP i pH 6.0 at varying concentrations of NaCl. ( b ) Comparison of the PRE profiles obtained at 0 mM (black) and 100 mM (blue) NaCl. Stars indicate the residues whose resonances disappear in the paramagnetic spectrum. The errors are s.d. The inset schematically depicts the experimental set-up, with the NMR-active protein coloured light blue, and the attached paramagnetic label indicated by the red sphere. ( c ) Ionic strength dependence of Γ 2 for several CL CcP residues. The errors are s.d. The red lines show the best fits to an exponential decay function with the decay rates of 28±4 (D140, r 2 =0.97), 36±6 (K183, r 2 =0.98) and 25±4 (N220, r 2 =0.98). 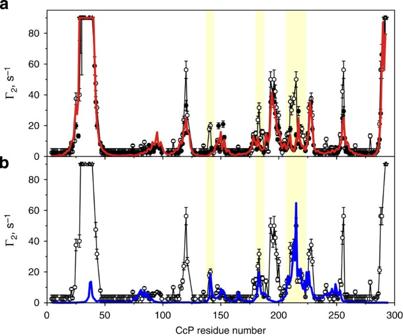Figure 7: PREs for the native non-covalent Cc–CcP complexes at low and high ionic strengths. (a,b) Intermolecular PREs for the backbone amide resonances of [D,15N] wt CcP interacting with Cc E88C-EDTA(Mn2+) in 20 mM NaPipH 6.0 and [NaCl]=0 mM (open symbols) or [NaCl]=100 mM (filled symbols). The high and low-salt samples contained 0.4 mM CcP and 1 or 3 equivalents of Cc, respectively. The high-salt data were taken from our previous work28. The red line inashows the Γ2values calculated for the combination of the high-affinity binding orientation and the encounter complex at [NaCl]=100 mM28. The blue line in (b) represents the PREs calculated for the combination of the dominant binding geometry and multiple, lowly populated protein–protein orientations constituting the low-affinity Cc–CcP complex (studied in this work) and corresponds to the red trace inFig. 3a. Several regions exhibiting differences between the high- and low-salt PRE profiles are highlighted. Full size image Figure 7: PREs for the native non-covalent Cc–CcP complexes at low and high ionic strengths. ( a , b ) Intermolecular PREs for the backbone amide resonances of [D, 15 N] wt CcP interacting with Cc E88C-EDTA(Mn 2+ ) in 20 mM NaP i pH 6.0 and [NaCl]=0 mM (open symbols) or [NaCl]=100 mM (filled symbols). The high and low-salt samples contained 0.4 mM CcP and 1 or 3 equivalents of Cc, respectively. The high-salt data were taken from our previous work [28] . The red line in a shows the Γ 2 values calculated for the combination of the high-affinity binding orientation and the encounter complex at [NaCl]=100 mM [28] . The blue line in ( b ) represents the PREs calculated for the combination of the dominant binding geometry and multiple, lowly populated protein–protein orientations constituting the low-affinity Cc–CcP complex (studied in this work) and corresponds to the red trace in Fig. 3a . Several regions exhibiting differences between the high- and low-salt PRE profiles are highlighted. Full size image Finally, to validate the location of the low-affinity binding site and assess the role of CcP residues D148 and D217 in the CL–Cc complex formation, we prepared two charge-reversal CL variants, in which either one or both of the aspartates are substituted by lysines. PRE NMR experiments with D217K and D148K/D217K CLs show that Cc-binding effects are greatly reduced in the former and even more so in the latter system ( Fig. 8 ). A large decrease is observed for the intermolecular PREs originating from both the dominant and minor CL–Cc forms, which can be attributed to changes in the electrostatic properties of CcP in the variant CLs. These results illustrate the importance of D148 and D217 residues for the low-affinity Cc–CcP complex formation and confirm that the negatively charged region of the CcP surface identified in the classic Brownian dynamics study [32] is indeed the location of the low-affinity binding site. 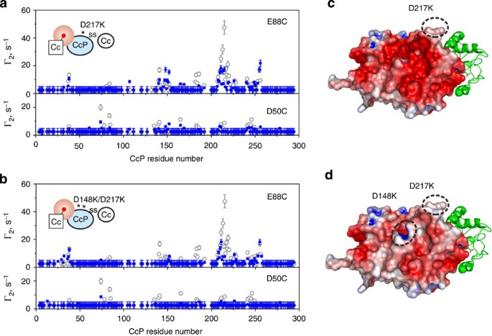Figure 8: PRE NMR analysis of the Cc interaction with the charge-reversal CcP–Cc CLs. (a,b) Intermolecular, CcP-observed PREs caused by the binding of the paramagnetically labelled E88C and D50C Cc to (a) D217K/V197C and (b) D148K/D217K/V197C [D,13C,15N] CcP–A81C Cc CLs. The measured PREs (blue symbols) are compared with those of the original, ‘wt’ CL (open symbols; also shown inFig. 3a). The errors are s.d. The insets schematically depict the experimental set-up, with the NMR-active protein coloured light blue, the attached paramagnetic label indicated by the red sphere and point mutations represented by asterisks. (c,d) The charge-reversal CLs with the molecular surface of CcP coloured by the electrostatic potential (from −5kBTin red to +5kBTin blue, calculated with APBS)57. The protein orientations are the same as inFig. 2h. The introduced mutations are indicated by dashed circles. All NMR samples contained 0.5 mM CL and 1 equivalents of Cc in 20 mM NaPipH 6.0. Figure 8: PRE NMR analysis of the Cc interaction with the charge-reversal CcP–Cc CLs. ( a , b ) Intermolecular, CcP-observed PREs caused by the binding of the paramagnetically labelled E88C and D50C Cc to ( a ) D217K/V197C and ( b ) D148K/D217K/V197C [D, 13 C, 15 N] CcP–A81C Cc CLs. The measured PREs (blue symbols) are compared with those of the original, ‘wt’ CL (open symbols; also shown in Fig. 3a ). The errors are s.d. The insets schematically depict the experimental set-up, with the NMR-active protein coloured light blue, the attached paramagnetic label indicated by the red sphere and point mutations represented by asterisks. ( c , d ) The charge-reversal CLs with the molecular surface of CcP coloured by the electrostatic potential (from −5 k B T in red to +5 k B T in blue, calculated with APBS) [57] . The protein orientations are the same as in Fig. 2h . The introduced mutations are indicated by dashed circles. All NMR samples contained 0.5 mM CL and 1 equivalents of Cc in 20 mM NaP i pH 6.0. Full size image ET properties of the low-affinity site In a broad range of biological systems, the ET rate constants are described by an exponential dependence on the distances between the redox centres [40] . Thus, to assess the ET properties of the low-affinity Cc–CcP complex, we analysed the separations between the haem group of Cc and two redox centres in CcP CpdI—the haem oxyferryl and W191 cation-radical ( Fig. 9 ). Judging from the large distances of 21 Å (haem–W191) and 22 Å (haem–haem), the dominant low-affinity binding geometry is inactive in the intermolecular ET. In contrast, the conformational ensemble constituting the minor form contains multiple, ET-competent protein–protein orientations with short haem–haem separations of <16 Å ( Fig. 9a ). Calculated from the edge-to-edge haem-to-haem distances in the four simulated ensembles (highlighted in Fig. 5a ) as the population-weighted average over all Cc–CcP orientations constituting the low-affinity complex, the ET rate ( k ET ) is found to be 1,324–2,343 s −1 . The overall average value of < k ET >=1,950±450 s −1 can be compared with the experimentally measured k ET =1,540±80 s −1 for direct haem–haem ET from the low-affinity domain in the 2:1 Cc–CcP complex [10] , [11] . As the high-affinity crystallographic orientation and the encounter state exhibit large separations between the prosthetic groups [7] , [28] , it appears that the low-affinity domain alone accounts for the measured haem–haem ET activity [8] , [9] , [10] , [11] . 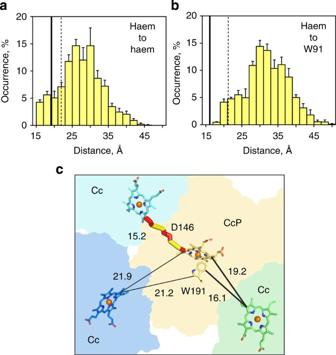Figure 9: ET properties of the low-affinity Cc–CcP complex. (a,b) Distributions of the edge-to-edge (a) haem–haem and (b) Cc haem–CcP W191 distances in the low-affinity complex. The values are averaged over the data sets highlighted inFig. 5a; the errors are s.d. The solid and dashed lines indicate the corresponding distances in the crystallographic orientation and the dominant low-affinity binding form, respectively. (c) Shortest edge-to-edge separations (in Å) among the redox centres in the high-affinity (thick lines) and low-affinity (thin lines and solid cylinders) complexes. Surface outlines of CcP and Cc in the crystallographic orientation are coloured yellow and green, while those of the dominant form and a representative ET active geometry of the low-affinity complex are in blue (bottom left) and cyan (top left), respectively. In the latter, the solid cylinders indicate the intermolecular ET pathway mediated by the covalent bonds (red) of the haem groups and the intervening CcP residue D146 and two through-space jumps (yellow). Figure 9: ET properties of the low-affinity Cc–CcP complex. ( a , b ) Distributions of the edge-to-edge ( a ) haem–haem and ( b ) Cc haem–CcP W191 distances in the low-affinity complex. The values are averaged over the data sets highlighted in Fig. 5a ; the errors are s.d. The solid and dashed lines indicate the corresponding distances in the crystallographic orientation and the dominant low-affinity binding form, respectively. ( c ) Shortest edge-to-edge separations (in Å) among the redox centres in the high-affinity (thick lines) and low-affinity (thin lines and solid cylinders) complexes. Surface outlines of CcP and Cc in the crystallographic orientation are coloured yellow and green, while those of the dominant form and a representative ET active geometry of the low-affinity complex are in blue (bottom left) and cyan (top left), respectively. In the latter, the solid cylinders indicate the intermolecular ET pathway mediated by the covalent bonds (red) of the haem groups and the intervening CcP residue D146 and two through-space jumps (yellow). Full size image The low-affinity complex studied here is adequately described by the ‘dynamic docking’ model of protein–protein interactions [41] , in which numerous, lowly populated Cc–CcP orientations contribute to the overall binding, but only a small number of these are ET active. Moreover, as illustrated by computational studies, which delineated the ET-competent regions of the Cc–CcP conformational space [42] and mapped out the ET coupling pathways to the protein surfaces [11] , the most ET active orientation is not necessarily the most thermodynamically stable. An example of a transient, ET-competent Cc–CcP orientation is given in Fig. 9c . With the haem-to-haem separation of 15 Å, this bound form is expected to be highly ET active. Indeed, analysis of the electronic tunnelling coupling with the model developed by Beratan et al. [43] identified the optimal ET pathway with the overall k ET rate of 3.6 × 10 5 s −1 . Originating at the conjugated π-system of the Cc haem, the pathway proceeds via two covalent bonds of the thioether-bound 4-ethylene substituent, followed by a through-space jump to the Oδ 2 atom of the CcP residue D146 and a travel along its Oδ 2 -C γ -C β -C α -C ′ covalent bonds, followed by another through-space jump to the CcP haem 1-methyl ( Fig. 9c ). Taken at the face value, the existence of the ET-competent binding geometries seems to contradict the findings of Erman and co-workers, who showed that covalent Cc–CcP complexes with the blocked high-affinity site—CcP(V197C)-Cc(A81C), primarily studied here, and CcP(E290C)-Cc(K73C), the first site-specific CL designed to probe the ET activity at the low-affinity site [24] —are inactive towards externally added Cc [29] . However, the fact that no enzyme turnover is observed while the haem-to-haem ET is feasible confirms that the catalytic cycle involves ET to the W191 cation-radical [1] , [2] , [29] and highlights the central role of this CpdI redox intermediate in the CcP function. In agreement with this conclusion, the low-affinity complex displays large separations between Cc haem and CcP W191 groups ( Fig. 9b ), indicating that it does not support the functionally relevant ET activity. This finding is also consistent with the studies of Hoffman and co-workers, as the ET observed in their flash photolysis experiments occurs directly between two haem groups, bypassing formation of W191 +· species [8] , [9] , [10] , [11] . While being of great academic interest, the low-affinity Cc–CcP binding appears to be irrelevant for the physiological function. As this interaction is abolished under the physiological, high ionic strength conditions, the cellular enzymatic activity of CcP relies solely on the intermolecular ET to CpdI W191 +· , taking place from the high-affinity, crystallographic Cc–CcP orientation. Protein samples Single-cysteine mutants of yeast Cc and CcP were prepared by site-directed mutagenesis using whole-plasmid synthesis PCR (WHOPS PCR) protocol [44] , starting from the DNA sequences coding for proteins with substituted native cysteine residues (T-5A/C102T Cc, referred to as the wt Cc [45] , and C128A CcP, prepared in a separate WHOPS PCR step). Charge-reversal CcP mutants D217K/V197C/C128A and D148K/D217K/V197C/C128A were prepared by additional WHOPS PCRs on the V197C/C128A CcP DNA template. All constructs were verified by DNA sequencing. Expression vectors for the wt proteins, Cc variants D50C, E66C and E88C, and the single-cysteine D32C Ub were prepared before [25] , [28] , [45] . The natural-abundance wt proteins and their single-cysteine variants, uniformly labelled [D, 15 N] wt and V197C/C128A CcP and 15 N-labelled wt Cc were produced in Escherichia coli and purified following published procedures [25] , [28] , [45] . The EDTA(Mn 2+ ) paramagnetic probe was attached via cysteine reaction with Mn 2+ complex of N-[S-(2-pyridylthio)cysteaminyl] ethylenediamine- N , N , N ′, N ′-tetraacetate monoamide (Toronto Research Chemicals), and the conjugated products were purified and characterized as described before [28] . The protein concentrations were calculated from the ultraviolet–visible spectra using the known extinction coefficients for the Soret band absorption maxima [14] , [25] , [45] . Complexes of the low-spin CcP(CN) and Cc (Fe 2+ ), mimicking the CpdI [46] , were studied throughout this work. All NMR samples were prepared in 20 mM NaP i pH 6.0 and contained 6 % D 2 O for the lock. Unless stated otherwise, the PRE measurements were conducted on 0.4 mM [D, 15 N] CcP–Cc CL and 1 equivalents of the Cc-EDTA(Mn 2+ ) (for the paramagnetic samples) or wt Cc (for the diamagnetic reference). The compositions of the samples used for the control experiments ( Figs 4 and 6 , 7 , 8 and Supplementary Fig. 5 ) are indicated in the corresponding figure legends. Synthesis of the disulfide CLs To obtain V197C CcP–A81C Cc and E290C CcP–K73C Cc CLs in high yield, we adopted the strategy of Otting and co-workers [23] , schematically shown in Supplementary Fig. 6 . First, to reduce the possible intermolecular disulfides, a relevant single-cysteine CcP variant was incubated with a 10-fold molar excess of DTT for 1 h at room temperature (RT) and then exchanged into 20 mM Tris-HCl 100 mM NaCl pH 8.0 on a HiTrap Desalting column (GE Healthcare), concomitantly removing the reductant. Second, the CcP—now bearing a free thiol group—was incubated with a 10-fold molar excess of 5,5′-dithiobis-(2-nitrobenzoate) [DTNB or Ellman’s reagent] for 1 h at RT, yielding the modified protein and the yellow-coloured TNB. The unreacted DTNB and the TNB product were removed on a desalting column, leaving the protein solution containing the CcP-TNB adduct. Third, a fivefold molar excess (relative to CcP) of the corresponding single-cysteine Cc variant was incubated with a 10-fold molar excess (relative to Cc) of DTT for 1 h at RT, exchanged into 20 mM Tris-HCl 100 mM NaCl pH 8.0 on a desalting column and combined with the CcP-TNB solution. The cross-linking reaction between the free thiol-bearing Cc and the TNB-activated CcP was carried out for 16–18 h at RT, yielding the desired disulfide-linked CcP–Cc heterodimer ( Supplementary Fig. 6 ). Finally, the protein CL was purified from the reaction mixture by ion-exchange chromatography and characterized by SDS–PAGE, ultraviolet–visible spectrophotometry and analytical size-exclusion chromatography ( Fig. 1 and Supplementary Figs 1 and 2 ). The analytical gel-filtration experiments were performed on an ENrich SEC 70 column (Bio-Rad) equilibrated in 20 mM sodium phosphate (NaP i ) 100 mM NaCl pH 6.0 and run at a flow rate of 0.5 ml min −1 . The CL samples were injected at a concentration of 0.25 mM. The Bio-Rad size-exclusion standard (a lyophilized mixture of molecular weight markers ranging from 1.35 to 670 kDa) was used to calibrate the column. Two charge-reversal CL variants, D217K/V197C and D148K/D217K/V197C CcP–A81C Cc containing the uniformly labelled [D, 13 C, 15 N] CcP, were prepared by the same procedure, yielding the desired pure products ( Supplementary Fig. 2 ). NMR experiments and data analysis The NMR experiments were conducted at 298 K on a Varian NMR Direct-Drive System 600 MHz spectrometer ( 15 N Cc-observed CL titrations) or an 800-MHz spectrometer equipped with either a RT or a salt-tolerant PFG-Z cold probe (all other experiments). The NMR data were processed in NMRPipe [47] and analysed in CCPN [48] . The assignments of the backbone amide resonances of [D, 15 N] CcP(CN) and 15 N Cc were taken from our earlier work [25] , [28] , [45] . For most of the CcP resonances in [D, 15 N] CcP–Cc CLs, the assignments could be transferred directly from the spectra of the free protein (see Results section above). The assignments of the charge-reversal CL variants, D217K/V197C and D148K/D217K/V197C CcP–A81C Cc containing the uniformly labelled [D, 13 C, 15 N] CcP, were verified by TROSY-selected, deuterium-decoupled 3D HNCA, HN(CO)CA, and out-and-back HN(CA)CB experiments. Except for several resonances of residues in and around the mutation sites, the 2D [ 1 H, 15 N] TROSY spectra of the variant CLs are virtually identical to that of the original [D, 15 N] V197C CcP–A81C Cc construct, indicating that the introduced point mutations do not perturb the CcP structure. NMR titrations were performed by incremental addition of the concentrated Cc stock solution (2.6–2.9 mM) to the CcP–Cc CL samples at the initial concentrations of 0.32–0.46 mM. At each increment, chemical shift perturbations of backbone amide resonances of either [D, 15 N] CcP–Cc CL or 15 N Cc were monitored in 2D [ 1 H, 15 N] correlation spectra. The titration curves were analysed with a two-parameter non-linear least-squares fit using a one-site binding model corrected for the dilution effect [46] . The average chemical shift perturbations were calculated as Δ δ =(Δ δ N 2 /50+Δ δ H 2 /2) 0.5 , where Δ δ N and Δ δ H are the chemical shift perturbations of the backbone amide nitrogen and proton, respectively, for a given protein residue. The 1 H Γ 2 PREs were obtained from two identical [ 1 H, 15 N] TROSY-selected heteronuclear single-quantum correlation experiments with the relaxation delay of 10 s run on the paramagnetic and diamagnetic samples. The resonances showing strong spectral overlap were excluded from the analysis. The ratios of the signal intensities were converted into the Γ 2 values, and the Γ 2 errors were propagated from the signal intensities and the spectral noise levels as described in our recent report [28] . Ensemble refinement against intermolecular PREs The coordinates of the Cc–CcP CL were taken from the X-ray structure (PDB ID 1S6V) [14] . Using the PRE data set obtained from the three EDTA(Mn 2+ ) conjugation sites (D50C, E66C and E88C Cc), the rigid-body simulated annealing refinement of the Cc–CL complex was carried out in Xplor-NIH [49] , [50] following the published procedure [34] . In brief, the position of the CL was fixed, and either a single or multiple copies of the Cc molecule were docked to minimize the energy function consisting of the PRE target term, van der Waals repulsion term to prevent atomic overlap between Cc and CL, and a weak radius-of-gyration restraint used to encourage intermolecular Cc–CL contacts [34] . Note that this procedure allows for the atomic overlap among Cc molecules constituting an ensemble, as well as among the Cc ensemble members and the Cc of the dominant bound form. To account for the mobility of the attached label, the calculated effects were averaged over an ensemble of 50 EDTA(Mn 2+ ) conformers generated by simulated annealing in torsion angle space [51] . As explained in the text, the relative populations of the two bound species, p 1 and p 2 , were varied in multiple refinement runs. As a rule, 100 independent calculations were performed in each run, and 50 solutions with lowest Q factors (see below) were selected for further analysis. To assess the agreement between the observed PREs and the PREs back-calculated from Cc ensembles generated in each run, we calculated the Q factor [34] (equation 1): where j =1–3 runs over the three EDTA(Mn 2+ ) attachment sites on Cc and is given by equation 2: where p 1 and p 2 are the total populations of the dominant and minor Cc–CL species, respectively, N is the ensemble size of the latter, Γ 2, ijk is the PRE from EDTA(Mn 2+ ) ( j ) back-calculated for the residue ( i ) of the Cc ensemble member ( k ), and Γ 2, ij is the PRE back-calculated from EDTA(Mn 2+ ) ( j ) for the residue ( i ) of Cc in the dominant form of the complex. ET rate calculations The rate constants for the intermolecular ET, k ET , were calculated from the edge-to-edge distances between the haem groups (equation 3) [40] : where k 0 =10 13 s −1 is the nuclear frequency, is the decay coefficient of the electronic coupling, r is the edge-to-edge distance between the redox centres, r 0 =3.6 Å is the van der Waals contact distance, Δ G is the free energy difference between reactant and product states, λ is the reorganization energy, k B is the Boltzmann constant and T is the temperature. The values of Δ G =−0.797 eV and λ =0.7 eV were taken from the literature [42] , [52] . As shown by Marcus and Sutin [53] and further confirmed by density functional theory calculations of the electron density distribution in the haem derivatives [54] , [55] , mixing of the t 2g -orbitals of the Fe center in Cc with the π*-orbitals of the porphyrin ring effectively extends the metal d -electron density to the porphyrin edge, which justifies the use of edge-to-edge distances in the ET analysis of the Cc–CcP system. The overall average < k ET > reported in the text was obtained from the k ET rates of the Cc–CcP complexes generated in four ensemble refinement runs with the smallest Q factors (highlighted in Fig. 5a ), calculated as population-weighted averages of the k ET values for individual protein–protein orientations in the 50 best Cc–CcP solutions. Alternatively, the k ET was derived from the analysis of the ET pathways (equation 4) [56] : where h is the Planck constant, T DA is the electronic donor-to-acceptor tunnelling coupling and the other symbols are the same as above. The T DA factor can be estimated using the Pathways model [43] , which treats electron tunnelling as a sequence of steps taking place through a covalent bond, a hydrogen bond, or the vacuum, and represents the T DA as the product of penalties for each step, equation 5 (ref. 56 ): where ɛ C =0.6 is the penalty for the covalent bond-mediated step; is the penalty for a through-space jump, where R S is the jump distance in Å; is the penalty for a hydrogen bond-mediated step, where R H is the hydrogen bond length in Å; and is the decay factor for the vacuum [56] . The search for the ET pathways and the T DA calculations were carried out with the Pathways plugin for the molecular visualization programme VMD [56] . In general, the k ET values calculated from the ET distances (equation 3) or obtained with the Pathways model (equations 4 and 5) in this work agreed to within a factor of two. Accession Codes: An NMR ensemble of 15 lowest-energy CL-Cc structures has been deposited in the Protein Data Bank under the code 2N18. How to cite this article: Van de Water, K. et al. The low-affinity complex of cytochrome c and its peroxidase. Nat. Commun. 6:7073 doi: 10.1038/ncomms8073 (2015).